A primase subunit essential for efficient primer synthesis by an archaeal eukaryotic-type primase Archaea encode a eukaryotic-type primase comprising a catalytic subunit (PriS) and a noncatalytic subunit (PriL). Here we report the identification of a primase noncatalytic subunit, denoted PriX, from the hyperthermophilic archaeon Sulfolobus solfataricus . Like PriL, PriX is essential for the survival of the organism. The crystallographic analysis complemented by sensitive sequence comparisons shows that PriX is a diverged homologue of the C-terminal domain of PriL but lacks the iron–sulfur cluster. Phylogenomic analysis provides clues on the origin and evolution of PriX. PriX, PriL and PriS form a stable heterotrimer (PriSLX). Both PriSX and PriSLX show far greater affinity for nucleotide substrates and are substantially more active in primer synthesis than the PriSL heterodimer. In addition, PriL, but not PriX, facilitates primer extension by PriS. We propose that the catalytic activity of PriS is modulated through concerted interactions with the two noncatalytic subunits in primer synthesis. DNA primases play a critical role in the initiation of DNA replication by synthesizing RNA primers on both the leading and lagging strands since DNA polymerases are incapable of de novo DNA synthesis. The majority of primases are classified into two major groups, that is, the bacterial DnaG-type primases and the more complex eukaryotic primases [1] . The bacterial primases are single subunit enzymes often found to interact with replicative DNA helicases [2] . The eukaryotic primases are a heterodimer of a small catalytic subunit (PriS or p48) and a large noncatalytic subunit (PriL or p58), which form a complex with DNA polymerase α (Pol α or p180) and the B subunit (p70) [3] . While PriS contains the active site and is responsible for catalysis in primer synthesis, PriL serves to regulate the activity of the primase and the transfer of a primer of 10 ∼ 15 nt in size to Pol α. Pol α recognizes the RNA primer and extends it, generating a RNA–DNA primer of 30 ∼ 40 nt in length [4] , [5] . No enzymatic activity has been assigned to the B subunit, but this protein is believed to play a regulatory role in the initiation of DNA replication [6] . Intriguingly, Archaea encode both types of DNA primase. It has been shown that the bacterial-type DnaG primase from the hyperthermophilic archaeon Sulfolobus solfataricus was active in primer synthesis [7] and interacted with MCM in vitro [8] . However, since archaeal DnaG was also found to be an integral part of the exosome [9] and dispensable for cell growth [10] , it is unclear if the protein is involved in primer synthesis during DNA replication. All experimentally characterized eukaryotic-type primases from Archaea are heterodimers of PriS and PriL homologues (PriSL) [10] , [11] , [12] , [13] . The archaeal primase complexes do not contain homologues of either Pol α or the B subunit. The archaeal PriSL has been suggested to function as the replicative primase. However, the archaeal primase substantially differs from its eukaryotic counterpart in many respects. Archaeal PriSL can catalyse de novo synthesis of both DNA and RNA products of various sizes up to several kilobases, depending on the template, primer extension and terminal nucleotidyl transfer using either ribonucleoside triphosphates (rNTPs) or deoxynucleoside triphosphates (dNTPs) as the substrates in vitro [14] , [15] . Also surprising is the observation that PriSL from S. solfataricus was nearly inactive in primer synthesis in vitro at high temperatures that are optimal for the growth of this organism [15] . Therefore, it remains unclear how the eukaryotic-type primase serves its proposed physiological role in Archaea. Here we report the identification of a primase noncatalytic subunit, denoted PriX, from S. solfataricus and show that PriX, PriS and PriL form a unique heterotrimeric primase complex capable of far more efficient primer synthesis than PriSL. A novel primase subunit from S. solfataricus Given that PriSL from S. solfataricus is known to possess unusual properties unexpected for the proposed role of the enzyme in DNA replication, we set out to determine if there existed additional proteins that might modulate the activity of PriSL. By using a co-immunoprecipitation assay, we found that an unknown protein was consistently immunoprecipitated with antibodies against PriS or PriL ( Fig. 1a ). Mass spectrometry identified this protein as the product of Sso0502, a gene that encodes a functionally uncharacterized polypeptide of 154 amino acid residues with a molecular mass of 18 kDa. No significant amino acid sequence similarity was detected between the product of Sso0502 and known primases or primase subunits or any other functionally characterized proteins when the PSI_BLAST programme was used to search the non-redundant protein sequence database at the NCBI (NIH, Bethesda) with default parameters. The only detected homologues were hypothetical proteins from many other archaea ( Supplementary Fig. 1 ). However, when one of these hypothetical protein sequences (GI|255513484 from Micrarchaeum acidiphilum ARMAN-2) was used as the query for a second round of PSI_BLAST, highly significant matches with numerous archaeal PriL homologues as well as eukaryotic PriL were detected. The HHpred search with the homologue of Sso0502 from Acidianus hospitalis (Ahos_0948) also identifies similarity with profile PRK09568 corresponding to DNA primase large subunit with the probability of ∼ 80%. 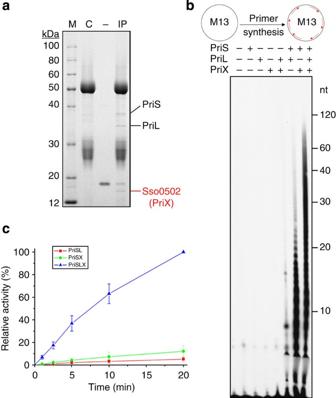Figure 1: PriX is a novel noncatalytic subunit of the primase fromS. solfataricus. (a) Co-immunoprecipitation of theS. solfataricuscell extract with anti-PriL antibodies. The cell extract was treated with DNase I/RNase A and subjected to immunoprecipitation with anti-PriL antibodies. C, no cell extract; IP, the immunoprecipitate; M, molecular weight markers; —, no anti-PriL antibodies. (b) Primer synthesis by PriS, PriL and PriX separately or in various combinations on M13 ssDNA with rNTPs as the substrates. PriX, PriS and/or PriL were incubated with M13 ssDNA in the standard assay mixture. A diagram depicting the template and the products (in red) is shown on top. (c) A time course of primer synthesis by PriSL, PriSX and PriSLX. PriSL, PriSX and PriSLX were incubated for indicated periods of time with dNTPs as the substrates on M13 ssDNA in the standard assay mixture. The relative activity corresponding to primer synthesis by PriSLX in a 20-min reaction is defined as 100%. Error bars represent s.d. of experimental triplicates. Figure 1: PriX is a novel noncatalytic subunit of the primase from S. solfataricus . ( a ) Co-immunoprecipitation of the S. solfataricus cell extract with anti-PriL antibodies. The cell extract was treated with DNase I/RNase A and subjected to immunoprecipitation with anti-PriL antibodies. C, no cell extract; IP, the immunoprecipitate; M, molecular weight markers; —, no anti-PriL antibodies. ( b ) Primer synthesis by PriS, PriL and PriX separately or in various combinations on M13 ssDNA with rNTPs as the substrates. PriX, PriS and/or PriL were incubated with M13 ssDNA in the standard assay mixture. A diagram depicting the template and the products (in red) is shown on top. ( c ) A time course of primer synthesis by PriSL, PriSX and PriSLX. PriSL, PriSX and PriSLX were incubated for indicated periods of time with dNTPs as the substrates on M13 ssDNA in the standard assay mixture. The relative activity corresponding to primer synthesis by PriSLX in a 20-min reaction is defined as 100%. Error bars represent s.d. of experimental triplicates. Full size image Orthologues of Sso0502 appear to be phylogenetically restricted to the phylum Crenarchaeota within the domain Archaea. According to the arCOG database and sequence similarity search results, all the species of the orders Sulfolobales and Acidilobales as well as some species of the order Desulfurococcales encode a single orthologue of Sso0502, whereas none of the species from the other two creanarchaeal orders, Thermoproteales and Fervidicoccales, encompass this gene ( Supplementary Table 1 ). Sso0502 was cloned and overexpressed in Escherichia coli , and the recombinant protein was purified (See Supplementary Information ). As shown in Fig. 1b , the purified protein alone was inactive in primase assays. PriS alone was equally inactive, as expected. Surprisingly, when the two proteins were both present in the assays, significant synthesis was observed, with products differing in size distribution from those characteristic of PriSL. This finding implies that the newly identified protein can at least partially substitute for the function of PriL. Notably, primer synthesis by PriSL in the presence of the Sso0502 product was over an order of magnitude ( ∼ 16-fold) more efficient than that in its absence, when the reaction was carried out at 55 °C, the optimal temperature for the primase activity of PriSL in vitro ( Fig. 1b,c ). Based on these results and those described below, we suggest that the product of Sso0502 is a novel noncatalytic subunit of the archaeal eukaryotic-type primase, and the protein is accordingly denoted PriX. We then attempted to determine the crystal structure of PriX. 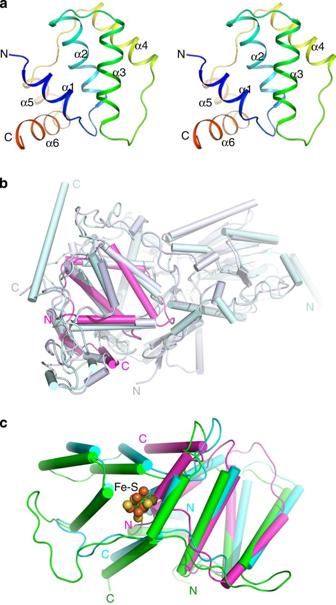Figure 2: The PriX structure is distantly related to the structure of eukaryotic PriL. (a) Three-dimensional structure of the N-terminally truncated PriX. α-helices are numbered. The N and C termini of the chain are labelled with letters. (b) Structural comparison of PriX (magentas) with cryptochrome 3 fromArabidopsis thaliana(PDB code 2IJG, Grey) andDrosophila melanogaster(6–4) photolyase (PDB code 3CVV, light blue). Helices and strands are shown as cylinders and arrows, respectively. (c) Structural comparison of PriX (magentas) with the N-terminal part of yeast PriL-CTD (PDB ID 3LGB, green) and human p58C (PDB ID 3Q36, cyan). Helices are shown as cylinders. Fe–S is shown as spheres. Because the full-length PriX protein failed to crystallize, we were only able to obtain crystals for a deletion mutant PriX protein containing amino acid residues 26–154 ( Supplementary Table 2 ). The crystal structure of the truncated protein was solved at 1.95 Å. The electron density for the entire truncated protein, except for its N-terminal portion (residues 26–54), was clear, permitting unambiguous placement of the residues. Presumably, residues 26–54 are in a flexible region. Residues 55–154 fold into a single domain containing 6 helices, which form a compact core stabilized by extensive hydrophobic interactions ( Fig. 2a and Supplementary Fig. 2 ). The overall structure of the PriX protein does not show strong similarity to any structures that are currently deposited in the PDB. However, a Dali search [16] identified weak structural similarity between PriX and cryptochrome proteins as well as many photolyases. Cryptochrome 3 from Arabidopsis thaliana (PDB code 2IJG) was the best match from the former family, with a Z score of 5.7 and the root mean square deviation (RMSD) of 3.2 Å for 88 matching C α positions [17] , and Drosophila melanogaster (6–4) photolyase (PDB code 3CVV) was the best match from the latter family, with a Z score of 5.4 and RMSD of 2.9 Å for 83 C α positions [18] ( Fig. 2b ). The truncated PriX also shows limited structural similarity (and ∼ 15% amino acid sequence similarity) to the N-terminal portion of the Fe–S domain at the C terminus of eukaryotic PriL (PriL-CTD), which contains amino acid residues known to be essential for the initiation of RNA primer synthesis by the primase [19] . For example, the match between PriX and yeast PriL (PDB code 3LGB) and that between PriX and human PriL (PDB code 3Q36) shows RMSDs of 3.28 Å for 79 C α positions and 3.61 Å for 83 C α positions, respectively [20] , [21] ( Fig. 2c ). A notable difference between PriX and its putative eukaryotic and archaeal homologues is that PriX lacks the iron–sulfur (Fe–S) cluster which is the signature of PriL-CTD. Recently, it has been shown that the N-terminal domain of the eukaryotic PriL-CTD shares a striking structural similarity with the active site-containing domain of the DNA photolyase/cryptochrome family of flavoproteins [20] . The combination of the results of sequence and structure comparisons suggests that PriX is a divergent homologue of PriL. Figure 2: The PriX structure is distantly related to the structure of eukaryotic PriL. ( a ) Three-dimensional structure of the N-terminally truncated PriX. α-helices are numbered. The N and C termini of the chain are labelled with letters. ( b ) Structural comparison of PriX (magentas) with cryptochrome 3 from Arabidopsis thaliana (PDB code 2IJG, Grey) and Drosophila melanogaster (6–4) photolyase (PDB code 3CVV, light blue). Helices and strands are shown as cylinders and arrows, respectively. ( c ) Structural comparison of PriX (magentas) with the N-terminal part of yeast PriL-CTD (PDB ID 3LGB, green) and human p58C (PDB ID 3Q36, cyan). Helices are shown as cylinders. Fe–S is shown as spheres. Full size image Evolution of primase subunits in Archaea To shed light on the origin of PriX, we carried out a detailed phylogenomic analysis of all archaeal primase subunits extracted from the arCOG database ( Supplementary Table 1 ). ArCOG04110 and arCOG03013 include the bona fide PriS and PriL, respectively, and are represented in almost all archaea. In addition, three arCOGs encompass divergent homologues of PriS and two arCOGs include distant homologues of PriL including PriX. Because PriS is the catalytic subunit of the primase and accordingly shows greater sequence conservation than PriL, we used the phylogenetic tree of PriS as the scaffold to examine the evolution of archaeal primase subunits ( Fig. 3 ). 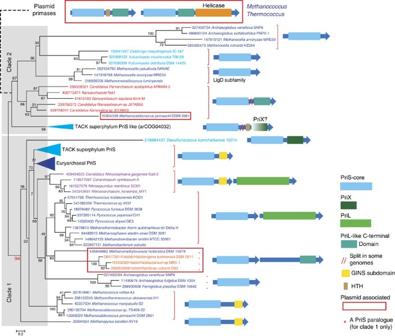Figure 3: Phylogenomic analysis of the archaeal PriS family. The maximum likelihood tree was reconstructed from a multiple sequence alignment that contained 112 sequences and 98 informative positions. Several branches are collapsed and shown as triangles denoted by the respective taxon name. The complete tree is available inSupplementary Fig. 3. The proteins are denoted by their GI numbers and species names. Colour code: Euryarchaeota, dark blue, with the exception of Halobacteria that are shown in orange;Crenarchaeota, light blue;Thaumarchaeota,Korarchaeota, purple; Nanoarchaea and other representative of small archaea, red. The conserved gene neighbourhoods and domain organizations are shown to the right of the tree for the respective branches. Homologous domains are shown by arrows of the same colour or shade. The dashed line shows the putative relationships between clade 2 and diverged PriL–PriS fusion protein encoded on euryarchaeal plasmids. Figure 3: Phylogenomic analysis of the archaeal PriS family. The maximum likelihood tree was reconstructed from a multiple sequence alignment that contained 112 sequences and 98 informative positions. Several branches are collapsed and shown as triangles denoted by the respective taxon name. The complete tree is available in Supplementary Fig. 3 . The proteins are denoted by their GI numbers and species names. Colour code: Euryarchaeota, dark blue, with the exception of Halobacteria that are shown in orange; Crenarchaeota , light blue; Thaumarchaeota , Korarchaeota , purple; Nanoarchaea and other representative of small archaea, red. The conserved gene neighbourhoods and domain organizations are shown to the right of the tree for the respective branches. Homologous domains are shown by arrows of the same colour or shade. The dashed line shows the putative relationships between clade 2 and diverged PriL–PriS fusion protein encoded on euryarchaeal plasmids. Full size image The phylogenetic tree of PriS consists of two major clades. Clade 1 includes the bona fide PriS that is often encoded in a previously described, conserved genomic context [22] ( Supplementary Fig. 3 ). In the archaea that encode PriS of Clade 1, the PriL subunit is often encoded by a stand-alone gene but in several genomes the priL gene forms a putative operon with priS ( Fig. 3 and Supplementary Fig. 3 ). Clade 1 also includes a distinct homologue of PriS that is encoded on plasmids in Halobacteria and Methanomethylovorans hollandica . The gene encoding this PriS homologue is adjacent to a gene for an uncharacterized protein (arCOG07894) that shares distant sequence similarity to PriL-CTD ( Supplementary Table 3 ). Most likely, this protein is a previously undetected, highly derived homologue of PriL that evolved independently of PriX. Interestingly, in Desulfurococcus kamchatkensis, PriX is fused to a diverged PriS homologue ( Fig. 3 ). Most sequences in Clade 2 are diverged PriS paralogues from both Euryarchaeota and the TACK ( Thaumarchaeota , Aigarchaeota , Crenarchaeota and Korarchaeota ) superphylum. Many of these PriS paralogues are annotated as hypothetical proteins. Several small archaea of the putative superphylum ( Nanoarchaea , Parvarchaeum , Nanosalina and others [23] ) encode a clearly identifiable fusion of Clade 2 PriS and the C-terminal region of PriL [22] that resembles the aforementioned PriS–PriX fusion in Desulfurococcus kamchatkensis ( Fig. 3 ). In most of the small archaea, this is the only primase-related gene detected in the genome, indicating that PriL-CTD can provide the functionality of the primase large subunit. Most of the TACK superphylum sequences in Clade 2 belong to a distinct family of PriS paralogues (arCOG04032) in which the PriS domain is fused to a helix-turn-helix domain followed by an uncharacterized domain that does not show significant similarity to other proteins ( Fig. 3 ). Secondary structure prediction for the latter domain yields a nearly perfect match to the PriX structure solved in this study ( Supplementary Fig. 4 ) although the domain in arCOG04032 proteins is considerably shorter than PriX. In some crenarchaeal genomes, this fusion is split into two genes ( Fig. 4a ). Furthermore, the phyletic pattern (presence/absence) of arCOG04032 largely complements the pattern of PriX. Taken together, these observations suggest that the C-terminal domain of arCOG04032 proteins is a derivative of PriL-CTD and thus a homologue of PriX. 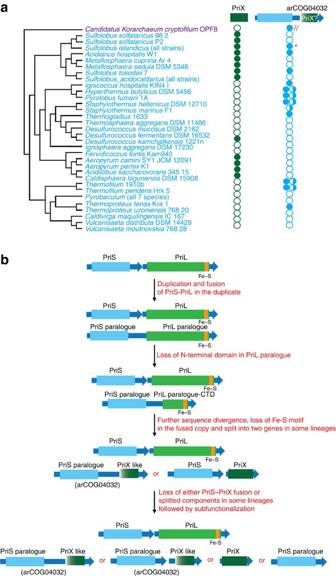Figure 4: Evolution of archaeal primase subunits. (a) Phyletic patterns of the PriX and arCOG04032 families (filled circles show presence and empty circles show absence, half-filled circles show truncated proteins of arCOG04032 family containing the C-terminal domain only) are superimposed over the phylogenetic tree of archaea. The tree topology is based on the phylogeny of concatenated ribosomal proteins35. The asterisk indicates that some strains ofSulfolobus islandicusencode either complete or split proteins or both. (b) A hypothetical scenario for PriX origin and evolution. Colour code, domain shapes and designations are the same as inFig. 3. Figure 4: Evolution of archaeal primase subunits. ( a ) Phyletic patterns of the PriX and arCOG04032 families (filled circles show presence and empty circles show absence, half-filled circles show truncated proteins of arCOG04032 family containing the C-terminal domain only) are superimposed over the phylogenetic tree of archaea. The tree topology is based on the phylogeny of concatenated ribosomal proteins [35] . The asterisk indicates that some strains of Sulfolobus islandicus encode either complete or split proteins or both. ( b ) A hypothetical scenario for PriX origin and evolution. Colour code, domain shapes and designations are the same as in Fig. 3 . Full size image Comparative genomic analysis of all archaeal genes and operons encoding primase subunits implies a complex evolutionary scenario. Considering the distribution of fused and separate PriS and PriL homologues among archaea, we speculate that duplication of an ancestral PriS–PriL operon, followed by gene fusion in one of the copies, occurred at an early stage in archaeal evolution ( Fig. 4b ). Compatible with this scenario, a recently identified primase from several thermococcal plasmids encompasses the fusion of PriS and PriL-CTD, with the Fe–S binding motif preserved [24] . Thus, PriX might have originated via fission of the ancestral PriS–PriL fusion gene, accompanied by partial degradation of the PriL moiety, such that only the PriL-CTD remained. Most of the arCOG04032 proteins seem to have also evolved in a similar manner ( Fig. 4b ). This evolutionary process apparently was accompanied by subfunctionalization of both the PriS and PriL paralogues. Furthermore, existence of other PriL-like proteins that have diverged beyond recognition by the current sequence comparison methods cannot be ruled out. PriX is essential for the growth of Sulfolobus Because PriX resembled PriL in enabling PriS to catalyse primer synthesis, we sought to determine if PriX was essential for the growth of the cell. We attempted to delete the PriX gene by using the marker insertion and target gene deletion method [25] ( Supplementary Fig. 5 ). However, no viable deletion mutants were obtained. A mutant propagation assay further established that PriX was essential for the survival of the Sulfolobus cell ( Supplementary Fig. 5c ). We also measured the intracellular levels of PriX along with PriS and PriL in S. solfataricus by quantitative immunoblotting. As shown in Supplementary Fig. 6 , the intracellular levels of PriX, PriL and PriS were largely unchanged during the early to mid-exponential growth phase, and the molar ratio of PriX, PriL and PriS was ∼ 1:2:13. However, the protein levels of both PriL and PriX decreased rapidly towards the end of the exponential growth phase and became undetectable in the death phase. In contrast, the intracellular concentration of PriS appeared to be stably maintained during the entire growth cycle. These results suggest that both PriL and PriX are involved in DNA replication, and PriS probably functions not only in DNA replication but also in other DNA transactions. PriX forms a heterotrimer with PriS and PriL Since PriSX was active in primer synthesis on M13 single-stranded DNA (ssDNA), we next examined the possibility of an interaction between PriS and PriX. As shown in Fig. 5a , PriX did not co-immunoprecipitate with PriS. Furthermore, no interaction between the two proteins was detected by surface plasmon resonance (SPR) or isothermal titration calorimetry (ITC). However, PriS and PriX were efficiently cross-linked with EDC in the presence of Sulfo-NHS, suggesting a weak interaction between the two proteins ( Fig. 5b ). Moreover, PriX co-immunoprecipitated with PriS in the presence of M13 ssDNA ( Fig. 5a ). Because PriS was unable to bind to ssDNA, whereas PriX strongly bound to ssDNA, as determined by EMSA under solution conditions similar to those used in the Co-immunoprecipitation assay ( Supplementary Fig. 7 ), it appears that DNA-bound PriX was capable of stably interacting with PriS. It was also noticed that PriX or PriS alone was cross-linked into oligomers. The ability of these proteins to oligomerize may contribute to the formation of higher-order primase complexes. 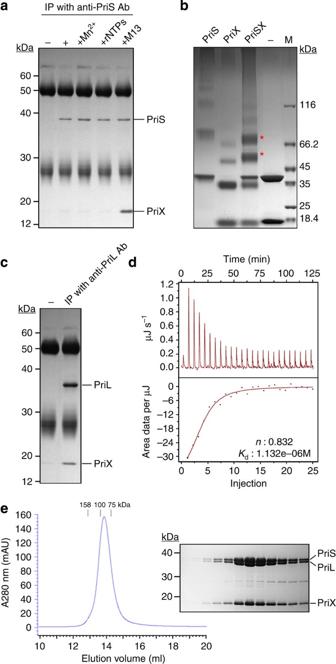Figure 5: Interactions between primase subunits. (a) Co-immunoprecipitation of PriS and PriX. PriS and PriX were mixed in the presence or absence of Mn2+, rNTPs or M13 ssDNA. Co-immunoprecipitation was performed with anti-PriS antibodies. (b) Chemical cross-linking between PriS and PriX. PriX and PriS were incubated with 10 mM EDC and 5 mM sulfo-NHS. The products of cross-linking between PriS and PriX are indicated by asterisks. (c) Co-immunoprecipitation of PriL and PriX. PriL and PriX were co-immunoprecipitated with anti-PriL antibodies. (d) Isothermal titration calorimetry of the interaction between PriL and PriX. PriL was titrated with PriX on the NANO-ITC 2G isothermal titration calorimeter. (e) Gel filtration analysis of the formation of the PriSLX heterotrimer. Recombinant PriX and PriSL were mixed, and the mixture was loaded onto a Superdex 200 column. Peak column fractions were analysed by SDS–PAGE. Figure 5: Interactions between primase subunits. ( a ) Co-immunoprecipitation of PriS and PriX. PriS and PriX were mixed in the presence or absence of Mn 2+ , rNTPs or M13 ssDNA. Co-immunoprecipitation was performed with anti-PriS antibodies. ( b ) Chemical cross-linking between PriS and PriX. PriX and PriS were incubated with 10 mM EDC and 5 mM sulfo-NHS. The products of cross-linking between PriS and PriX are indicated by asterisks. ( c ) Co-immunoprecipitation of PriL and PriX. PriL and PriX were co-immunoprecipitated with anti-PriL antibodies. ( d ) Isothermal titration calorimetry of the interaction between PriL and PriX. PriL was titrated with PriX on the NANO-ITC 2G isothermal titration calorimeter. ( e ) Gel filtration analysis of the formation of the PriSLX heterotrimer. Recombinant PriX and PriSL were mixed, and the mixture was loaded onto a Superdex 200 column. Peak column fractions were analysed by SDS–PAGE. Full size image On the other hand, PriX readily co-immunoprecipitated with PriL, indicating a stable interaction between the two proteins ( Fig. 5c ). Stoichiometry measurement by ITC revealed a molar ratio of one for the PriL–PriX complex ( Fig. 5d ). Given that PriL-CTD contains a Fe–S cluster, that is essential for the initiation of primer synthesis in Eukarya [19] , in its C-terminal domain, we tested whether this domain was involved in the PriL–PriX interaction. We found that a PriL deletion mutant lacking the C-terminal domain (PriLΔCTD) lost the ability to interact with PriX ( Supplementary Fig. 8a ). Consistent with this finding, a hybrid protein containing the C-terminal domain of PriL (PriL-CTD) fused to glutathione S-transferase (GST) (GST-PriL-CTD) interacted with PriX, indicating that the PriL-CTD was involved in the PriL–PriX interaction ( Supplementary Fig. 8b ). Deletion analysis shows that an N-terminally truncated PriX mutant protein-containing residues 41–154 resembled full-length PriX in enhancing primer synthesis by PriS ( Supplementary Fig. 9a ). Furthermore, like the full-length protein, the truncated PriX co-immunoprecipated with PriS in the presence of M13 ssDNA ( Supplementary Fig. 9b ). However, the truncated protein was unable to co-immunoprecipitate with PriL ( Supplementary Fig. 9c ), suggesting that the N terminus of PriX is involved in the interaction of this protein with PriL. We then sought to determine if PriS, PriL and PriX were able to form a heterotrimer. All three proteins were mixed, and the mixture was subjected to gel filtration. The three proteins co-eluted as a heterotrimer with a molar ratio of 1:1:1, as indicated by the elution volume and by quantification of each protein from the peak fractions on a Coomassie blue-stained SDS–PAGE gel ( Fig. 5e ). Notably, deletion of the C-terminal domain of PriL resulted in dissociation of PriX from the heterotrimer ( Supplementary Fig. 8c ). Based on these results, we conclude that PriS, PriL and PriX exist as a heterotrimer in solution, and the Fe–S-containing C-terminal domain of PriL serves an important role in stabilizing the complex. PriX and PriL bind template DNA differently Template DNA binding by PriX, PriL, PriS and their complexes was compared by electrophoretic mobility shift assays (EMSA) ( Supplementary Fig. 7 ). While PriS was unable to bind to an ssDNA, both PriX and PriL bound to the DNA under the experimental conditions. Notably, the two noncatalytic subunits displayed distinctly different binding patterns although both had similar binding affinities ( K d :0.05 ∼ 0.1 μM), as judged by the amount of the protein required to retard half of the input DNA. PriX produced clearly resolvable shifts, whereas PriL generated smears, which presumably resulted from dissociation of the protein from the DNA during electrophoresis. PriSL was also able to form large complexes with the DNA. Interestingly, binding of the ssDNA by PriSLX ( K d : ∼ 0.05 μM) not only was tighter than that by PriSL ( K d : 0.1 ∼ 0.2 μM) but also exhibited a pattern, which appears to combine the characteristics of binding by the two noncatalytic subunits. These results indicate that both PriL and PriX are involved in the binding of the heterotrimeric primase to the template. Both PriSX and PriSLX differ from PriSL in primer synthesis To determine how PriX might affect the ability of PriS and PriSL to synthesize primers, we compared PriSX and PriSLX with PriSL in primase assays at different temperatures in the presence of either rNTPs or dNTPs ( Fig. 6a–c ). The three complexes displayed several distinct differences in primer synthesis. First, both PriSX and PriSLX were substantially more active in primer synthesis than PriSL on an M13 ssDNA template. Second, the size distribution of the products synthesized by PriSX or PriSLX differed from that for PriSL. Oligonucleotides synthesized by PriSL showed a wider distribution in size than those synthesized by PriSX and PriSLX. Third, the three complexes showed similar temperature dependences, with the optimal activity at 45–55 °C. However, PriSLX appeared to have a broader range of temperatures for significant primase activity than PriSX. Notably, PriSLX was capable of efficient primer synthesis at 75 °C, a temperature at which S. solfataricus thrives. By contrast, no measurable primer synthesis with either PriSL or PriSX was observed at this temperature. Given the above differences between the three complexes, it appears that, in the PriSLX complex PriL and PriX modulated the catalytic activity of PriS in a coordinated manner. 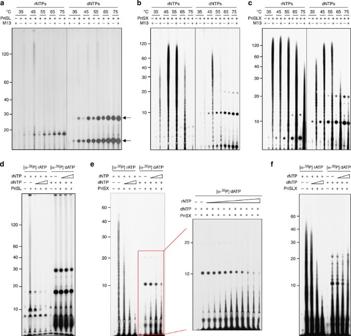Figure 6: Both PriSX and PriSLX differ from PriSL in primer synthesis. (a–c) Effects of temperature and substrates on the primase activity of PriSL, PriSX and PriSLX. PriSL, PriSX or PriSLX was incubated with M13 ssDNA for 30 min in the presence of indicated substrates and at indicated temperatures. Bands indicated by an arrow (a) are short products that PriSL was able to synthesize in the absence of a template. Recently, the two spots were identified as dAMP-glycerol (the lower band) and dAMP-Tris (the higher band)36. The exposure time for the gel inawas about three times as long as those for the gels inb,c. (d–f) Incorporation of dNMPs or rNMPs by PriSL, PriSX and PriSLX in the presence of rNTPs or dNTPs, respectively. Primase was incubated with M13 ssDNA at 55 °C (PriSL), 65 °C (PriSX) or 75 °C (PriSLX) in the presence of a fixed amount (10 μM) of radiolabelled dNTPs and an increasing amount (0, 1, 10 and 100 μM) of unlabelled rNTPs or a fixed amount (10 μM) of radiolabelled rNTPs and an increasing amount (0, 1, 10 and 100 μM) of unlabelled dNTPs. For PriSX, incorporation of dNMPs was also tested in the presence of rNTPs at increased concentrations (0, 0.25, 0.5, 1, 2, 5, 10, 20, 50, 100 and 200 μM) (panel to the right ofFig. 2e). Figure 6: Both PriSX and PriSLX differ from PriSL in primer synthesis. ( a – c ) Effects of temperature and substrates on the primase activity of PriSL, PriSX and PriSLX. PriSL, PriSX or PriSLX was incubated with M13 ssDNA for 30 min in the presence of indicated substrates and at indicated temperatures. Bands indicated by an arrow ( a ) are short products that PriSL was able to synthesize in the absence of a template. Recently, the two spots were identified as dAMP-glycerol (the lower band) and dAMP-Tris (the higher band) [36] . The exposure time for the gel in a was about three times as long as those for the gels in b , c . ( d – f ) Incorporation of dNMPs or rNMPs by PriSL, PriSX and PriSLX in the presence of rNTPs or dNTPs, respectively. Primase was incubated with M13 ssDNA at 55 °C (PriSL), 65 °C (PriSX) or 75 °C (PriSLX) in the presence of a fixed amount (10 μM) of radiolabelled dNTPs and an increasing amount (0, 1, 10 and 100 μM) of unlabelled rNTPs or a fixed amount (10 μM) of radiolabelled rNTPs and an increasing amount (0, 1, 10 and 100 μM) of unlabelled dNTPs. For PriSX, incorporation of dNMPs was also tested in the presence of rNTPs at increased concentrations (0, 0.25, 0.5, 1, 2, 5, 10, 20, 50, 100 and 200 μM) (panel to the right of Fig. 2e ). Full size image A steady-state kinetic analysis of primer synthesis by PriSL, PriSX and PriSLX was performed on M13 ssDNA at 55 °C ( Table 1 and Supplementary Fig. 10 ). The K m values of both PriSX and PriSLX for dNTPs or rNTPs were in a micromolar range. On the other hand, the velocity of primer synthesis by PriSL increased almost linearly with increasing concentrations (up to at least 2 mM) of either dNTPs or rNTPs and, therefore, neither K m nor V max for PriSL could be determined under the assay conditions. This is not surprising since the rate of primer synthesis by PriSL from S. solfataricus was reported to increase with an increasing concentration of dNTPs, and the V max was not reached even at a dNTPs level of 43 mM [15] . However, the K m of PriSL for rNTPs was measurable in the previous study [15] . Based on our results, it is estimated that the affinities of PriSX and PriSLX for dNTPs and rNTPs were at least 2 orders of magnitude higher than those of PriSL. Furthermore, the affinity of PriSLX ( K m : 3.2±0.75 μM) for rNTPs was approximately five times as high as that of PriSX ( K m : 14.1±3.4 μM), whereas the two complexes were similar in affinity for dNTPs ( K m values of 5.42±1.1 and 8.75±0.6 μM for PriSLX and PriSX, respectively). The in vitro rate of rNMP incorporation by PriSLX was twice as high as that by PriSX. So the catalytic efficiency ( k cat / K m ) of PriSLX was about 1 order of magnitude higher than that of PriSX in primer synthesis with rNTPs as the substrates. PriSL was ∼ 30- and ∼ 300-fold less efficient in catalytic performance than PriSX and PriSLX, respectively. Interestingly, when dNTPs were used as the substrates, PriSX appeared to be sensitive to substrate inhibition ( K i : 244.8±8.6 μM) as the velocity of incorporation started to decrease at >50 μM dNTPs ( Supplementary Fig. 10b ). PriSLX was ∼ 3 orders of magnitude more catalytically efficient than PriSL. Furthermore, PriSLX was more than twice as efficient in incorporating rNMPs as in incorporating dNTPs. Table 1 Kinetic parameters for primer synthesis. Full size table We also examined primer synthesis by the three primase complexes in the presence of both dNTPs and rNTPs. The reaction entailed both the formation of the first dinucleotide and the subsequent extension of the first dinucleotide by using either dNTPs or rNTPs. It has been reported that incorporation of ribonucleotides by PriSL was strongly inhibited by dNTPs, whereas the incorporation of deoxyribonucleotides by this heterodimer was only slightly affected by rNTPs present at a large molar excess [13] , [14] . The same observation was made on PriSL in this study ( Fig. 6d ). To determine if PriSX and PriSLX would behave similarly to PriSL, we incubated the primase complexes with a fixed amount of radiolabelled dNTPs and an increasing amount of unlabelled rNTPs, or a fixed amount of radiolabelled rNTPs and an increasing amount of unlabelled dNTPs. We found that rNMP incorporation by both PriSX and PriSLX was strongly inhibited by the addition of dNTPs, whereas dNMP incorporation by the two complexes was not inhibited by the addition of rNTPs, as observed in the case of PriSL ( Fig. 6e,f ). Notably, however, incorporation of dNMPs by the two primase complexes was affected differently by rNTPs. PriSX was inefficient in incorporating dNMPs in the presence of dNTPs alone, but the incorporation was significantly enhanced by the addition of rNTPs even at low rNTPs/dNTPs molar ratios (for example, 0.1) ( Fig. 6e ), suggesting that initial polymerization during primer synthesis by PriSX occurred preferably with rNTPs and was then followed by the efficient incorporation of dNTPs. By comparison, PriSLX was able to incorporate dNMPs readily in the absence of rNTPs ( Fig. 6c ), and incorporation of dNMPs by the heterotrimer was not drastically affected by the presence of rNTPs even at a large molar excess (for example, an rNTPs/dNTPs ratio of 10) ( Fig. 6f ). Therefore, PriSX initiated primer synthesis more efficiently with rNTPs than with dNTPs. PriL but not PriX enhances primer extension by PriS To test the ability of PriSLX, PriSL and PriSX to extend a preformed primer, we prepared a primed template by annealing a 32 P-labelled 40-nt oligoribonucleotide to M13 ssDNA (R40/M13). As shown in Fig. 7a , PriSX was no more active than PriS, which was barely able to extend the primer in the presence of either rNTPs or dNTPs, indicating that PriX was not able to facilitate primer extension by PriS. In contrast, both PriSL and PriSLX produced longer extension products than that synthesized by PriS, especially in the presence of rNTPs. As a control, no significant terminal transfer by any of the primase complexes or subunits was observed on R40 under the experimental conditions. Thus, PriL enhanced the ability of PriS to extend a template primer. 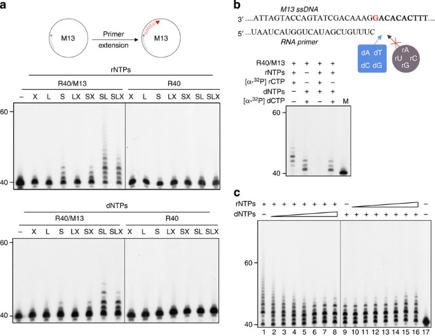Figure 7: PriSL is essential for primer extension. (a) RNA primer extension by PriS, PriL and PriX separately or in various combinations in the presence of indicated substrates. PriS, PriL and PriX were incubated individually or in various combinations with a32P-labelled 40-nt RNA primer annealed to M13 ssDNA (R40/M13) or R40 for 15 min at 75 °C. A diagram depicting the reaction is shown on the top. (b) RNA primer extension by PriSL in the presence of both dNTPs and rNTPs. PriSL was incubated with an unlabelled 40-nt RNA primer annealed to M13 ssDNA in the presence of unlabelled rNTPs or dNTPs containing either [α-32P]rCTP or [α-32P]dCTP. (c) RNA primer extension by PriSL in the presence of dNTPs or rNTPs. PriSL was incubated with32P-labelled R40/M13 in the presence of a fixed amount (100 μM) of rNTPs and an increasing amount (0, 2, 5, 10, 20, 100, 500 and 1,000 μM) of dNTPs or a fixed amount (100 μM) of dNTPs and an increasing amount (0, 2, 5, 10, 20, 100, 500 and 1,000 μM) of rNTPs. Figure 7: PriSL is essential for primer extension. ( a ) RNA primer extension by PriS, PriL and PriX separately or in various combinations in the presence of indicated substrates. PriS, PriL and PriX were incubated individually or in various combinations with a 32 P-labelled 40-nt RNA primer annealed to M13 ssDNA (R40/M13) or R40 for 15 min at 75 °C. A diagram depicting the reaction is shown on the top. ( b ) RNA primer extension by PriSL in the presence of both dNTPs and rNTPs. PriSL was incubated with an unlabelled 40-nt RNA primer annealed to M13 ssDNA in the presence of unlabelled rNTPs or dNTPs containing either [α- 32 P]rCTP or [α- 32 P]dCTP. ( c ) RNA primer extension by PriSL in the presence of dNTPs or rNTPs. PriSL was incubated with 32 P-labelled R40/M13 in the presence of a fixed amount (100 μM) of rNTPs and an increasing amount (0, 2, 5, 10, 20, 100, 500 and 1,000 μM) of dNTPs or a fixed amount (100 μM) of dNTPs and an increasing amount (0, 2, 5, 10, 20, 100, 500 and 1,000 μM) of rNTPs. Full size image To determine the substrate preference of PriSL in primer extension, we performed assays on unlabelled R40/M13 in the presence of both rNTPs and dNTPs including either [α- 32 P]rCTP or [α- 32 P]dCTP ( Fig. 7b ). Extension products were detected in the presence of either rNTPs including [α- 32 P]rCTP or dNTPs including [α- 32 P]dCTP, as expected. Surprisingly, however, although labelled products of various sizes were synthesized in the presence of a dNTP label supplemented with unlabelled rNTPs at an rNTPs/dNTPs ratio of 1, no labelled products were detected in the reaction containing a rNTP label and unlabelled dNTPs at the same rNTPs/dNTPs ratio. Apparently, dNTPs outcompeted rNTPs for incorporation during primer extension by PriSL. To verify this observation, primer extension was measured on labelled R40/M13 in the presence of both dNTPs and rNTPs at rNTPs/dNTPs molar ratios from 50 ( Fig. 7c , lane 2) to 0.1 ( Fig. 7c , lane 8). The addition of dNTPs in the presence of large excess amounts of rNTPs (rNTPs/dNTPs ratio of 10) resulted in a switch of the pattern of the products from the one obtained in the presence of rNTPs alone to the one observed in the presence of dNTPs alone, as judged by the difference between the mobilities of oligoribonucleotides and oligodeoxyribonucleotides of the same size in the sequencing gel. By contrast, extension of the primer with dNMPs was not affected by the addition of rNTPs even at an rNTPs/dNTPs molar ratio of >5 ( Fig. 7c , lanes 15 and 16). In agreement with this finding, we found in a kinetic experiment that the affinity of PriSL for dGTP ( K m : 0.06±0.01 μM) was over two fold higher than that for rGTP ( K m : 0.14±0.04 μM), and the catalytic efficiency of the primase heterodimer for dGMP incorporation was 3.6-fold higher than that for rGMP incorporation ( Supplementary Fig. 11 ). These results reveal that PriSL prefers dNTPs over rNTPs during primer extension. In this report, we identify a novel primase noncatalytic subunit, denoted PriX, from S. solfataricus . Genetic analysis shows that PriX is essential for the growth of S. solfataricus . Highly conserved PriX homologues are present in many members of the phylum Crenarchaeota . Detailed sequence analysis combined with structural analysis of a truncated PriX protein shows that PriX is homologous to the C-terminal domain of archaeal and eukaryotic large primase subunits (PriL-CTD). The structure of the eukaryotic PriL-CTD consists of two α-helical domains joined at the interface by a Fe–S cluster [20] . PriX corresponds to the larger, N-terminal α-helical domain, which represents the most conserved portion of the eukaryotic PriL-CTD and bears a striking structural similarity to the active site region of the photolyase/cryptochrome protein family [20] , [21] . Thus, PriX is a truncated derivative of PriL. Moreover, in several archaeal genomes, we detected additional putative derived homologues of PriL-CTD that seem to have evolved independently of PriX. Notably, PriX and some of the other PriL derivatives lack the Fe–S cluster that is highly conserved among bona fide PriL-CTDs. The potential structural role of the Fe–S cluster in the noncatalytic primase subunit might be fulfilled by intramolecular interactions within PriX and other PriL derivatives. PriX, PriL and PriS form a stable heterotrimer with a 1:1:1 stoichiometry. In this complex, PriX appears to interact primarily with the C-terminal domain of PriL because deletion of this domain resulted in the loss of PriX from the complex. Eukaryotic PriL-CTD is believed to function in RNA primer synthesis via its Fe–S domain by assisting PriS in the simultaneous binding of the two initial ribonucleotides and by concomitantly promoting dinucleotide base-pairing with template DNA at the initiation site [20] . In addition, the eukaryotic PriL-CTD is probably involved in coordinating the transfer of the nascent oligoribonucleotide from the core primase to Pol α [26] . Archaeal PriL proteins show substantial sequence divergence from their eukaryotic orthologues. The structure of the archaeal PriL-CTD, which contains a conserved Fe–S cluster, has not yet been solved. Surprisingly, a dimeric complex of PriS and PriL lacking the CTD was only slightly less active than the wild-type heterodimer in primer synthesis in vitro , suggesting that the Sulfolobus PriL-CTD is not essential for the primase activity of PriSL and that the archaeal PriL-CTD might differ from the eukaryotic PriL-CTD in function [27] . This finding, along with the observation that PriSL is much less efficient than PriSX in primer synthesis, raises the possibility that PriL-CTD primarily serves to bind and position PriX in such a way that it can contribute to the initiation of primer synthesis upon interacting with PriS on the template DNA. Kinetic experiments reveal that PriSX differs strikingly from PriSL in primer synthesis. While primer synthesis by PriSX and PriSLX exhibited the typical Michaelis–Menten-type kinetics, with a micromolar K m for dNTPs or rNTPs, the rate of nucleotide incorporation by PriSL increased almost linearly with the substrate concentrations under the assay conditions. The mechanistic basis for this difference is unclear. Given the observations that PriSX initiated primer synthesis more efficiently with rNTPs than with dNTPs, synthesized shorter products than PriSL and tended to terminate primer extension upon incorporation of dNTPs in vitro , it appears to be well suited for a role in the initial stage of primer synthesis, when a short RNA primer is synthesized de novo . The influence of PriX on primer synthesis by PriS was clearly demonstrated in the catalytic properties of the heterotrimeric PriSLX complex. Primer synthesis by PriSLX was readily terminated even when rNTPs were present in a large excess over dNTPs. Therefore, primers synthesized by PriSLX are most likely terminated at the 3’ end with a short stretch of DNA. Based on these results, we propose that the primer synthesis in S. solfataricus proceeds as follows. PriS, PriL and PriX exist as a stable heterotrimer in solution. Binding to a DNA template alters and stabilizes the interaction between PriX and PriS, initiating the synthesis of a primer using preferentially rNTPs. Once the nascent primer reaches a certain length, conformational changes in PriSLX may occur, permitting the primer to be handed over from PriX to PriL via the interaction between PriX and the C-terminal Fe–S domain of PriL. PriSL subsequently carries out limited primer extension by incorporating primarily dNTPs, generating an RNA–DNA hybrid primer. The primer is then elongated by the replicative DNA polymerase. This hypothesis implies that a single catalytic subunit (PriS) is shared during the two steps of primer synthesis, and the activity of PriS is modulated through its highly coordinated interaction with two different noncatalytic subunits (PriX and PriL). Given that PriX is essential for the growth of S. solfataricus , it is unclear how archaea lacking PriX carry out primer synthesis. Phylogenomic analysis described in this paper revealed several other PriL derivatives that seem to have evolved independently of PriX, and more such proteins could remain to be identified given their high sequence divergence. Thus, a functional counterpart of PriX might exist in many, if not most, archaea. Further studies on primases of various archaeal origins are expected to shed light on the evolution of the archaeal-eukaryotic primer synthesizing machinery and its catalytic mechanism. Crystallization and structure determination Crystals of truncated PriX (residues 26–154) were grown, and diffraction data were collected at Rigaku CCD944+. The data sets were indexed, integrated and scaled in space group P2 1 2 1 2 1 , and the crystals diffracted X-rays to 1.95 Å. See Supplementary Methods for further details. Co-immunoprecipitation and mass spectrometry Cells from an exponentially growing S. solfataricus culture (OD 600 of ∼ 0.4) were harvested and resuspended in lysis buffer (50 mM Tris-HCl, pH 6.8, 150 mM NaCl, 0.1 mM DTT and 10% (v/v) glycerol). The cells were lysed either with 0.5% Triton X-100 or by sonication, and centrifuged at 30,000 g for 20 min at 4 °C. The supernatant was incubated for 30 min at 4 °C with DNase I (100 U) and RNase A (100 U). Immunoprecipitation with indicated antibodies and subsequently with protein A beads was performed according to the manufacturer’s instruction (Clontech). The antibodies were prepared in rabbit with purified recombinant proteins as the antigens. The immunoprecipitates were resolved by SDS–PAGE, and the gel was stained with Coomassie brilliant blue G250. Proteins of interest were recovered from the gel and identified by liquid chromatography-tandem mass spectrometry. To detect protein–protein interactions, two tested proteins (10 μg each) were co-immunoprecipitated as described above. Rabbit antibodies against PriX, PriS or PriL were employed in the assays. Primase assays The standard reaction mixture (10 μl) contained 50 mM MES-NaOH, pH 6.5, 10 mM MnCl 2 , 100 μg ml −1 BSA, 10 μM rNTP(s) or dNTP(s) including [α- 32 P]rNTP or [α- 32 P]dNTP, respectively, 250 ng M13mp18 and 1.5 μM primase. After incubation at indicated temperatures for 30 min or indicated times, the mixtures were stopped by the addition of an equal volume of stop buffer (98% deionized formamide, 10 mM EDTA and 0.025% bromophenol blue), boiled for 3 min, cooled rapidly on ice and subjected to electrophoresis through a 20% polyacrylamide gel containing 8 M urea in 1 × TBE. The gel was exposed to X-ray film or analysed by using an ImageQuant Storm PhosphorImager (Amersham Biosciences). Primer extension assays The reaction mixture (10 μl) contained 50 mM MES-NaOH, pH 6.5, 10 mM MnCl 2 , 100 μg ml −1 BSA, 100 μM rNTP(s) or dNTP(s) including [α- 32 P]rCTP or [α- 32 P]dCTP, respectively, 2 nM primed template R40/M13 and 0.5 μM primase. For assays in which a 32 P-labelled primer annealed to the template ( 32 P-R40/M13) was used, radioactive nucleoside triphosphates were omitted. After incubation for 15 min at 75 °C, reaction products were extracted with phenol/chloroform/isoamyl alcohol, mixed with an equal volume of the gel loading buffer, boiled for 3 min and cooled rapidly on ice. Aliquots were subjected to electrophoresis in a 20% polyacrylamide gel containing 8 M urea in 1 × TBE, and the gel was exposed to X-ray film. Kinetic assays The standard assay mixture for primer synthesis contained 1.5 μM primase, 250 ng M13mp18, various amounts of dNTPs including [α- 32 P]dGTP or rNTPs including [α- 32 P]rGTP in 50 mM MES-NaOH, pH 6.5, 10 mM MnCl 2 and 100 μg ml −1 BSA. The reaction was performed for 30 min at 55 °C. Aliquots of the reaction solution were quenched with an equal volume of stop solution. Products were separated on a 20% polyacrylamide gel containing 8 M urea in 1 × TBE. The gel was analysed by using an ImageQuant Storm PhosphorImager. Known amounts of [α- 32 P]dGTP or [α- 32 P]rGTP were spotted on the gel to allow the construction of a standard curve for quantification of the reaction products. Data were subjected to nonlinear regression analysis with Michaelis–Menten steady-state kinetics or substrate inhibition kinetics. The standard reaction mixture for primer extension contained 10 nM primase, various concentrations of nucleotides and 250 nM primed template R25/T85 ( Supplementary Table 4 ) with R25 labelled at the 5′ end with 32 P in 50 mM MES-NaOH, pH 6.5, 10 mM MnCl 2 and 100 μg ml −1 BSA. Reactions were performed for 15 min at 75 °C and quenched by the addition of an equal volume of stop solution. Samples were subjected to eletrophoresis in 15% polyacrylamide gel containing 8 M urea in 1 × TBE. The gel was processed, and the data were analysed as described above. Analytical gel filtration Samples (200 μl) of the proteins were loaded on a Superdex 200 column (GE Healthcare), and eluted with 50 mM Tris-HCl, pH 7.0, and 150 mM NaCl. The column was calibrated with a set of gel filtration markers that included tyroglobulin, ferritin, BSA and ovalbumin. Column fractions were analysed by SDS–PAGE. Chemical cross-linking Samples of PriS and PriX, each at 8 μM, were cross-linked for 30 min at 23 °C with 10 mM EDC (Pierce) in the presence of 5 mM sulfo-NHS (Pierce) in 25 mM MES-NaOH, pH 6.5, and 150 mM NaCl. The cross-linking products were resolved by SDS–PAGE and the gel was stained with Coomassie brilliant blue G250. Isothermal titration calorimetry PriX and PriL were dialysed against 20 mM Tris-HCl, pH 7.0, 150 mM NaCl and 5% glycerol. PriL (10 μM) was titrated with PriX (120 μM) at 25 °C on the NANO-ITC 2G isothermal titration calorimeter (TA Instruments). Calorimetric data were analysed by nonlinear regression using a single-site binding model with Nanoanalyse Data Analysis. Sequence analysis The sequences related to PriS, PriL and PriX protein families from 168 completely sequenced archaeal genomes and information about the respective arCOGs were extracted from the arCOG database [28] (updated in February 2014). Additional sequences for deeply branched archaea related to Nanoarchaea were retrieved from the non-redundant protein sequence database at the NCBI using PSI_BLAST [29] programme, with the Nanoarchaeal sequence as the query (GI: 490715471). A single representative from closely related groups of archaeal genomes was chosen for further analysis (see the complete list of archaeal genomes selected for the analysis in the Supplementary Table 1 ). Iterative profile searches with the PSI_BLAST [29] programme with the cut-off e-value of 0.01, and composition-based statistics and low complexity filtering turned off were used for sequence searches. The HHpred programme with default parameters was used for detection of distant sequence similarity [30] . Multiple sequence alignments were built using the MUSCLE [31] programme. Protein secondary structure was predicted using the JPred programme [32] . For gene neighbourhood analysis, three upstream and downstream genes were extracted from the respective genome records. For each neighbouring gene, the Pfam identifiers and COG numbers as well as corresponding annotations were assigned using the RPS_BLAST programme and the Conserved Domain Database (CDD) [33] . The FastTree programme [34] with default parameters (JTT evolutionary model and discrete gamma model with 20 rate categories) was used for phylogenetic tree reconstruction. Accession codes : Atomic coordinates and structure factors of the truncated PriX crystallographic structure have been deposited in the Protein Data Bank with accession codes 4WYH. How to cite this article : Liu, B. et al. A primase subunit essential for efficient primer synthesis by an archaeal eukaryotic-type primase. Nat. Commun. 6:7300 doi: 10.1038/ncomms8300 (2015).